Conjugated organic framework with three-dimensionally ordered stable structure and delocalized π clouds Covalent organic frameworks are a class of crystalline organic porous materials that can utilize π–π-stacking interactions as a driving force for the crystallization of polygonal sheets to form layered frameworks and ordered pores. However, typical examples are chemically unstable and lack intrasheet π-conjugation, thereby significantly limiting their applications. Here we report a chemically stable, electronically conjugated organic framework with topologically designed wire frameworks and open nanochannels, in which the π conjugation-spans the two-dimensional sheets. Our framework permits inborn periodic ordering of conjugated chains in all three dimensions and exhibits a striking combination of properties: chemical stability, extended π-delocalization, ability to host guest molecules and hole mobility. We show that the π-conjugated organic framework is useful for high on-off ratio photoswitches and photovoltaic cells. Therefore, this strategy may constitute a step towards realizing ordered semiconducting porous materials for innovations based on two-dimensionally extended π systems. Porous materials are ubiquitous in nature. Cell membranes, honeycombs, foams, sponges, volcanic rocks and concretes are common everyday examples, which consist of organic or inorganic three-dimensional network architectures and inherent structural pores. They find important applications in science and technology, ranging from hydrogen storage to catalysis [1] . At the molecular level, available porous skeletons are composed of aluminosilicate [2] , silica [3] , metal-organic frameworks [4] or organic networks [5] . Among organic skeletons, covalent organic frameworks (COFs) [6] , [7] , [8] , [9] , [10] utilize π–π-stacking interactions for the crystallization of organic polygon sheets to form layered frameworks and ordered pores. Therefore, COFs comprise a unique class of materials made from purely organic composites and linkages, which create periodically ordered nanoscopic pores through crystallization of covalently linked organic polygons [6] , [7] , [8] , [9] , [10] , [11] , [12] , [13] , [14] , [15] , [16] , [17] , [18] , [19] , [20] , [21] , [22] , [23] , [24] , [25] , [26] , [27] , [28] , [29] . Two-dimensional (2D) COFs are characterized by their periodically ordered columnar π arrays and aligned one-dimensional nanochannels [6] , [7] , [8] , [9] , [10] , [11] , [12] , [13] , [14] , [15] , [16] , [17] , [18] , [19] , [20] , [21] , [22] , [23] , [24] , [25] , [26] , [27] , [28] , [29] , which are rarely available in other molecular architectures. In addition to traditional boronate [7] , [8] , [9] , [11] , [13] , [14] , [15] , [17] , [18] , [19] , [20] , [21] , [23] , [25] , [26] , [27] and boroxine [7] , [10] linkages, hydrazone [12] , imine [16] , [22] and squaraine [24] linkages have been developed for the solvothermal synthesis of COFs. Especially, covalent triazine frameworks synthesized by the trimerization of nitrile units under ionothermal conditions in the presence of molten salt such as ZnCl 2 [30] , [31] , [32] , [33] , [34] or by microwave reaction [35] offer a molecular platform to construct carbon nitride-conjugated networks, which exhibit outstanding properties and functions. Exploration of new linkage and new reaction for the synthesis of COFs is a key to achieve the further advancement of functional porous materials. By virtue of their three-dimensional orderings at the atomic scale, 2D COFs have shown a great potential to perform core functions in organic electronics such as light emission [9] , [10] , charge transfer and separation [23] , [27] , and semiconduction [9] , [10] , [17] , [19] , [20] , [21] , [23] , [26] , [28] , [29] . However, typical COFs lack intrasheet π-conjugation and chemical stability, which significantly limit their practical utility. To address this shortcoming, a chemically stable yet fully π-conjugated COF is highly desirable. Such a framework with three-dimensionally ordered chain alignment may provide a solution for the long-standing daunting challenges in semiconducting polymer technology [36] , [37] , [38] . In this context, conjugated microporous polymers (CMPs) are a class of organic porous polymers that inherently combine π conjugation and porosity and provide unique structures and have been explored previously in applications [39] , [40] , [41] , [42] , [43] , [44] , [45] , [46] , [47] , [48] , [49] , [50] , [51] , [52] , [53] , [54] , [55] , [56] . However, CMPs are amorphous materials that lack intra- and intermolecular alignments and are difficult to develop as a molecular motif for designing ordered π-conjugated polymer systems [41] , [45] , [54] . A conjugated polymer that combines permanent porosity and structural 3D ordering such as 2D COFs remains to be well explored. Here we report a chemically stable, electronically conjugated 2D COF with topologically designed wire frameworks and open nanochannels. The conjugated COF permits inherently periodic ordering of conjugated chains in all three dimensions and displays a striking combination of physical properties: chemical stability, extended π-delocalization, ability to host guest molecules and hole mobility. We show that this fully π-conjugated COF is useful for high on-off ratio photoswitches and photovoltaic cells. Our COFs introduce a new strategy and direction in the quest for high-performance-conjugated polymers and may pave a way for innovations and applications in fields from organic electronics to energy storage, and fuel cells. 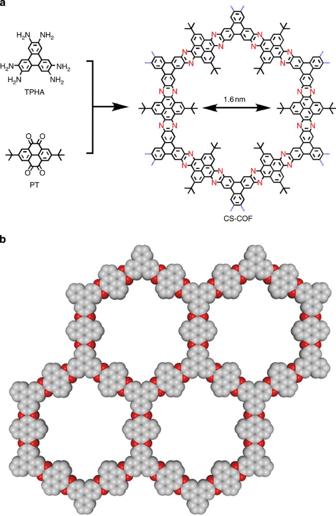Figure 1: Chemical structure. (a) Schematic representation of the synthesis of CS-COF. The dotted blue lines on the periphery imply the extension of periodic structures. (b) Graphic representation of one-layer-conjugated skeleton (a 2 × 2 CPK net; grey: carbon, red: nitrogen,tert-butyl groups and H atoms are omitted for clarity). The COF is mesoscopic platelets with lengths and widths extended to 1 μm and thicknesses ranged from 20 to 100 nm. Synthesis and characterization Figure 1 shows the structure of a chemically stable, electronically π-conjugated COF (CS-COF; CS stands for conjugated and stable). We selected C 3 -symmetric triphenylene hexamine (TPHA) [57] and C 2 -symmetric tert -butylpyrene tetraone (PT) [58] as building blocks for the topological ring fusion reaction and prepared the crystalline phenazine-linked CS-COF in isolated yields of 86–90% under solvothermal conditions. The tert -butyl side groups in PT were employed for enhancing the solubility of monomer. As an amorphous analogue, phenazine-linked-CMP Aza-CMPs that were synthesized using ionothermal conditions in the presence of AlCl 3 as a molten salt at 300–500 °C have been explored for supercapacitive energy storage [50] . CS-COF was unambiguously characterized using various analytical methods ( Supplementary Figs S1–S3 ). Elemental analysis confirmed that its C, H and N contents were 83.68%, 5.12% and 10.55%, respectively, which were close to the theoretical values of 84.02%, 5.09%, and 10.89%, respectively, expected for an infinite sheet. Fourier-transform infrared (FT IR) spectra indicated the formation of phenazine linkages with characteristic bands at 1,519, 1,431, and 1,354 cm –1 ( Fig. 2a , red curve). However, the vibration bands due to the NH 2 group of TPHA (3,384 and 3,313 cm –1 ) and the C=O unit of PT (1,676 cm –1 ) disappeared ( Fig. 2a , black curves), whereas those due to the C–H bonds of triphenylene ring at 3,044 and 1,623 cm –1 and the tert -butyl group at 2,923 and 2,852 cm –1 remained. Solid-state 1 H nuclear magnetic resonance (NMR) displayed two signals at δ =7.7 and 1.8 p.p.m., which are assignable to the protons of the aromatic rings and tert -butyl groups, respectively ( Fig. 2b ). Solid-state 13 C cross-polarization magic angle spinning (CP/MAS) NMR produced three signals at δ =140, 128 and 33 p.p.m., which are assignable to the aromatic carbons connected to the tert -butyl groups, other aromatic carbons and tert -butyl carbons, respectively ( Fig. 2c ). Moreover, solid-state 15 N CP/MAS NMR spectroscopy revealed that CS-COF consists of nitrogen atoms that appear at δ =–67.6 p.p.m., which corresponds to the nitrogens of phenazine and has an S/N ratio similar to that of the reported sample ( Fig. 2c ) [59] . Field-emission scanning electron microscopy revealed platelet objects ( Supplementary Fig. S1a ). Atomic force microscopy (AFM) revealed that the lengths and widths of these objects were ~1 μm ( Supplementary Fig. S1b ), and their thicknesses ranged from 10 to 200 nm, with most having thicknesses of 40–80 nm. High-resolution transmission electron microscopy (HR TEM) showed that the COF consists of parallel-aligned 2D sheets ( Fig. 3a ), which indicates a highly ordered alignment and corresponds to the (001) facet as seen in the X-ray diffraction (XRD) profile ( Fig. 4a ), whereas Fig. 3b reveals the porous texture of CS-COF. A broad absorbance across the ultraviolet and visible regions that further extend to near-IR regions indicates extended π cloud delocalization in the skeleton ( Supplementary Fig. S2 ). Frontier molecular orbitals support the delocalization of π clouds over the 2D skeleton ( Supplementary Fig. S3 ). Figure 1: Chemical structure. ( a ) Schematic representation of the synthesis of CS-COF. The dotted blue lines on the periphery imply the extension of periodic structures. ( b ) Graphic representation of one-layer-conjugated skeleton (a 2 × 2 CPK net; grey: carbon, red: nitrogen, tert -butyl groups and H atoms are omitted for clarity). The COF is mesoscopic platelets with lengths and widths extended to 1 μm and thicknesses ranged from 20 to 100 nm. 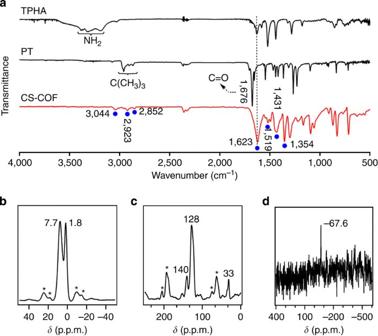Figure 2: FT IR and NMR spectral profiles. (a) FT IR spectrum of CS-COF (red curve) and the monomers TPHA and PT (black curves). Filled blue circles are a guide to the eye. (b–d) Solid-state1H (b),13C (c),15N (d) NMR spectra of CS-COF (*sidebands). Full size image Figure 2: FT IR and NMR spectral profiles. ( a ) FT IR spectrum of CS-COF (red curve) and the monomers TPHA and PT (black curves). Filled blue circles are a guide to the eye. ( b – d ) Solid-state 1 H ( b ), 13 C ( c ), 15 N ( d ) NMR spectra of CS-COF (*sidebands). 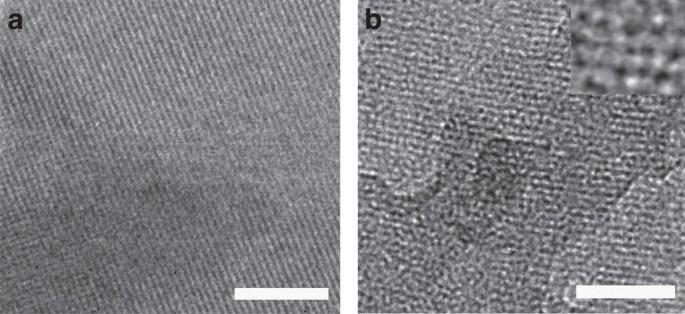Figure 3: Microscopic images. HR TEM images of (a) parallel-aligned sheets (scale bar, 5 nm) and (b) pores (scale bar, 20 nm). Full size image Figure 3: Microscopic images. HR TEM images of ( a ) parallel-aligned sheets (scale bar, 5 nm) and ( b ) pores (scale bar, 20 nm). 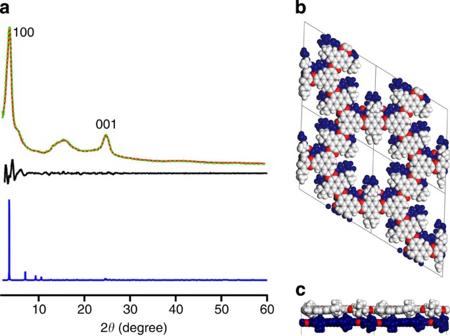Figure 4: XRD pattern and crystalline structure. (a) XRD profile of CS-COF (red curve), the Pawley-refined pattern (green curve) and their difference (black curve). XRD patterns were simulated using the P1 space group with the 0.8-Å-slipped AA-stacking mode (blue curve). (b,c) One pore structure of the 0.8-Å-slipped AA-stacking mode along thez- (b) andy- (c) axes. Full size image Figure 4: XRD pattern and crystalline structure. ( a ) XRD profile of CS-COF (red curve), the Pawley-refined pattern (green curve) and their difference (black curve). XRD patterns were simulated using the P1 space group with the 0.8-Å-slipped AA-stacking mode (blue curve). ( b , c ) One pore structure of the 0.8-Å-slipped AA-stacking mode along the z - ( b ) and y - ( c ) axes. Full size image Crystalline structural resolution Figure 4a shows the XRD pattern of the crystalline CS-COF (red curve). We tested the chemical stability of CS-COF by dispersing the sample in different solvents for 24 h and found that there was no change in their XRD patterns ( Supplementary Fig. S4 ). Their crystalline structure remained intact in organic solvents, such as methanol, benzene, CHCl 3 and hexane, irrespective of their polarity, in addition to aqueous HCl and NaOH solutions (1 M). We resolved the crystalline structure using XRD measurements in conjunction with structural simulations. The strongest peak at 2 θ of 3.7° can be assigned to the (100) facet of a regularly ordered hexagonal lattice. The peak at 25° is assignable to the (001) facet (π stacking), which is as also evident by the parallel alignment of 2D sheets in the TEM images. These results suggest that CS-COF has periodicities in all three dimensions. The XRD peaks of COFs are usually broad as a result of less-ordered edges in particles and/or a possible conformational fluctuation of 2D layers at mesoscopic scale [6] . One may notice that this peak broadness and intensity decrement of XRD signals becomes more explicit when flexible side groups are introduced to the pore walls of COFs. In this case, although the kernel part of particles is highly crystalline as shown by the HR TEM images, the side groups prevent the growth of large crystalline particles and give rise to more amorphous edges. Although the amorphous edge parts cannot be precisely estimated by XRD, the edge parts did not interfere the layered structure as shown by the HR TEM images. Similar broadened peaks were reported for boronate-linked COFs (for example, COF-16Å, COF-14Å and COF-11Å) with amorphous side groups on the pore walls [15] , [18] . Moreover, COF-11Å with propyl chains on the walls exhibited a broad halo peak at 2 θ from 12° to 22°. This peak appears significantly as the alkyl chain becomes longer from methyl to ethyl and propyl groups [15] . In the present CS-COF, the tert -butyl side groups cause a same effect on the XRD pattern. Considering the above points, characterization of the crystalline structure of CS-COF was performed using a combination of techniques including (1) the Pawley refinement to confirm the XRD peak assignment, (2) density functional tight-binding (DFTB) calculations to produce optimal structure of layered unit cell and (3) utilization of the optimal unit cell to reconstruct the XRD pattern. Figure 4a shows the Pawley-refined XRD curve (dotted green curve), which has a small difference (black curve) between the experimental curve (red curve). Together with small R wp (2.36%) and R p (1.85%) values, this result supports that the above peak assignments of (100) and (001) facets are correct. Theoretical simulations To quantitatively evaluate the interlayer-stacking interactions, we employed the self-consistent charge DFTB method including the Lennard–Jones (LJ) dispersion. Supplementary Table S1 summarizes the results. The 0.8-Å slipped AA-stacking mode (atomic coordinates are given in the Supplementary Table S2 ) has a total crystal-stacking energy of 110.20 kcal mol –1 per unit cell, which is considerably greater than those of the eclipsed AA stacking (29.01 kcal mol –1 ) and the staggered AB modes (74.15 kcal mol –1 ). These significant energy differences confirm that the slipped AA-stacking mode is superior to the other modes. This result is reasonable because the eclipsed stacking structure causes the clash of tert -butyl groups between neighbouring layers. The 0.8-Å slipped AA-stacking mode yields an XRD pattern ( Fig. 4a , blue curve) that reproduces the (100) and (001) facets. Figure 4b,c illustrates the one pore unit of the 0.8-Å slipped AA-stacking mode. The energy levels of the highest occupied molecular orbit (HOMO) and the lowest unoccupied molecular orbit calculated with the self-consistent charge DFTB method were –5.70 and –3.69 eV, respectively ( Supplementary Table S1 ). 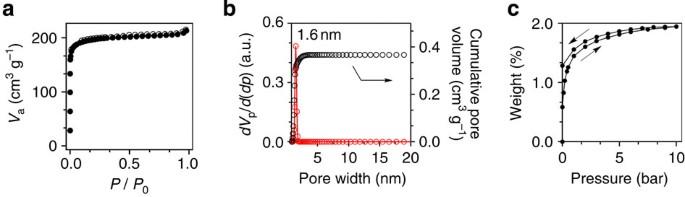Figure 5: Porous structure and gas adsorption. (a) Nitrogen adsorption (black circle) and desorption (open circle) isotherm profiles of CS-COF measured at 77 K. The sorption process is reversible and results in typical type I curves. (b) Pore size distribution (red open circle) and cumulative pore volume (black open circle) obtained by non-local density functional theory modelling on the N2adsorption curve. (c) Hydrogen sorption isotherm curves at 77 K. Gas adsorptions Figure 5a shows nitrogen sorption isotherm curves of CS-COF measured at 77 K. CS-COF is microporous showing a type I curve and a significant uptake in the low-pressure region ( P / P 0 <0.1). The Brunauer–Emmett–Teller surface area is as high as 776 m 2 g –1 and the pore volume is 0.34 cm 3 g –1 . Figure 5b shows the pore size distribution profile, which confirms that there is only one type of pore that accounts for the porosity. The pore width derived from the sorption curve using the non-local density functional theory method is 1.6 nm, which is consistent with the size measured from the crystalline structure. Figure 5c exhibits that CS-COF can adsorb hydrogen with a good capacity of 1.94 wt% at 77 K and 10 bar. Figure 5: Porous structure and gas adsorption. ( a ) Nitrogen adsorption (black circle) and desorption (open circle) isotherm profiles of CS-COF measured at 77 K. The sorption process is reversible and results in typical type I curves. ( b ) Pore size distribution (red open circle) and cumulative pore volume (black open circle) obtained by non-local density functional theory modelling on the N 2 adsorption curve. ( c ) Hydrogen sorption isotherm curves at 77 K. Full size image We investigated the inherent charge carrier mobility using the flash photolysis time-resolved microwave conductivity method [17] , [19] , [20] , [21] . Excitation under Ar with a 355-nm pulsed laser at a photon density of 2.6 × 10 16 photons cm –2 yielded a φ Σ μ value ( φ : the photocarrier generation quantum yield; Σ μ : the sum of charge carrier mobilities) of 0.50 cm 2 V –1 s –1 ( Fig. 6a ). When measured under SF 6 (electron quencher), CS-COF exhibited the same φ Σ μ value, which suggests that holes are the major charge carriers in the conduction. To determine the yield of charge carriers, the time-of-flight transient conductivity was integrated at different bias voltages ( Fig. 6b ). The number of charge carriers estimated by extrapolation of the bias at 0 V was 3.2 × 10 15 , yielding φ =12% ( φ =number of charge carriers/number of photons (2.6 × 10 16 )). Therefore, CS-COF is a high-rate hole-conducting framework with exceptional mobility of 4.2 cm 2 V –1 s –1 , which is ranked among the top-class hole-transporting organic semiconductors [7] , [20] , [29] . 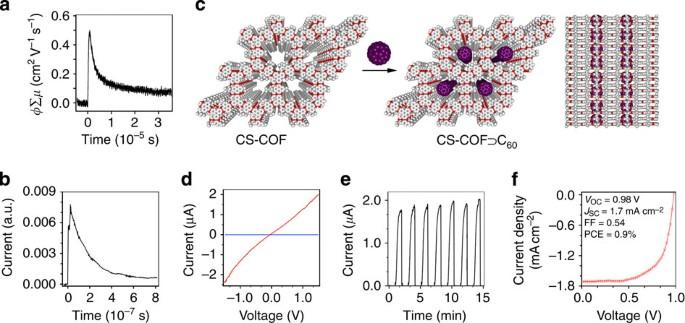Figure 6: Carrier mobility and photoelectric properties. (a) Conductivity transient using flash photolysis time-resolved microwave conductivity methods on excitation with a 355-nm laser pulse. (b) Time-of-flight transient current integration for CS-COF with a 355-nm laser pulse at a power of 34 mJ cm–2per pulse. (c) Schematic representation of synthesis of CS-COF⊃C60 by sublimed crystallization of fullerenes in the open one-dimensional channels (white: carbon; red: nitrogen; purple: fullerene). A side view of CS-COF⊃C60 is also shown. (d) I–V curve of a 50-nm-thick CS-COF⊃C60/PMMA film sandwiched between Al and Au electrodes at bias voltages ranging from –1.5 to 1.5 V in air at 25 °C. (e) Photocurrent switching at a bias voltage of 1.5 V in air at 25 °C, with repetitive light on-off actions on the 50-nm-thick CS-COF⊃C60/PMMA film. (f) J–V curve of the photovoltaic cell under irradiation with air mass 1.5 conditions (VOC=0.98 V,JSC=1.7 mA cm–2, FF=0.54). Figure 6: Carrier mobility and photoelectric properties. ( a ) Conductivity transient using flash photolysis time-resolved microwave conductivity methods on excitation with a 355-nm laser pulse. ( b ) Time-of-flight transient current integration for CS-COF with a 355-nm laser pulse at a power of 34 mJ cm –2 per pulse. ( c ) Schematic representation of synthesis of CS-COF ⊃ C60 by sublimed crystallization of fullerenes in the open one-dimensional channels (white: carbon; red: nitrogen; purple: fullerene). A side view of CS-COF ⊃ C60 is also shown. ( d ) I–V curve of a 50-nm-thick CS-COF ⊃ C60/PMMA film sandwiched between Al and Au electrodes at bias voltages ranging from –1.5 to 1.5 V in air at 25 °C. ( e ) Photocurrent switching at a bias voltage of 1.5 V in air at 25 °C, with repetitive light on-off actions on the 50-nm-thick CS-COF ⊃ C60/PMMA film. ( f ) J–V curve of the photovoltaic cell under irradiation with air mass 1.5 conditions ( V OC =0.98 V, J SC =1.7 mA cm –2 , FF=0.54). Full size image In addition to the functions of gas storage, CS-COF allows for complementary functionalization using the microporous space to crystallize counterpart fullerene molecules that can merge extended π conjugation with bicontinuous order into a donor–acceptor system (CS-COF ⊂ C 60 ). Figure 6c shows the synthesis and top and side views of CS-COF ⊃ C 60 . Because of the slipped AA stacking and the presence of bulky tert -butyl groups on the walls, the nanochannels accommodate only one C 60 molecule in the cross-section. The presence of C 60 in the pores of CS-COF is revealed by the drastic decrease in nitrogen gas sorption ( Supplementary Fig. S5 ). The strong diffraction peaks in the XRD pattern assignable to C 60 indicate that the C 60 molecules are crystallized in CS-COF ( Supplementary Fig. S6 ). The C 60 content in CS-COF ⊃ C 60 is ~25 wt% as revealed by both elemental and thermal gravimetric analysis (TGA; Supplementary Fig. S7 ), suggesting a peapod-like encapsulation of C 60 molecules in the pores. We fabricated 1 × 1 cm 2 sandwiched devices with a configuration of Al/poly(methyl methacrylate (PMMA; as a glue): CS-COF ⊃ C 60 /Au. Indeed, on irradiation from the Au side with the visible light (>400 nm) of a xenon lamp, CS-COF ⊃ C 60 was photoconductive, displaying a rapid response to light irradiation. The devices were optimized with various PMMA contents and film thickness ( Supplementary Fig. S8 ), and the best on-off ratio (5.9 × 10 7 ) was obtained for a device with a film thickness of 50 nm and a PMMA content of 50 wt%. In this case, the photocurrent was as high as 2.0 μA ( Fig. 6d , red curve), whereas the dark current was 0.029 pA (blue curve) at a bias voltage of 1.5 V. The films of CS-COF ⊃ C 60 allow multiple rounds of on-off switching without a loss of performance at room temperature ( Fig. 6e ). Photoswitches have been targeted for high-speed optical computing and data processing, whereas high on-off performance and visible light control are the requirements for such materials. For this purpose, a variety of materials have been developed using ferrocene-doped PMMA, diarylethene, spiropyrans, zinc oxide nanowires, poly(phenylene ethynylene) nanowires, polymer-coated carbon nanotubes and single-crystal phthalocyanine ribbons as active layers; however, they exhibit quite low on-off ratios (<10 3 ) (ref. 60 ). On the other hand, the best photoswitches (1 × 10 6 ) thus far reported have to work by ultraviolet light [60] . Remarkably, CS-COF is superior to all other COFs including hole-conducting PPy-COF (8 × 10 4 ) (ref. 10 ) and NiPc-COF (150) (ref. 17 ), electron-conducting NiPc-BTBA COF (60) (ref. 19 ), and ambipolar-conducting ZnP-COF (5 × 10 4 ) (ref. 20 ) and 2D D–A COF (1.3 × 10 4 ) (ref. 21 ). The high photocarrier generation efficiency (12%) and ordered bicontinuous structure may explain the exceptional on-off ratio. Along these lines, we investigated the possibility of using CS-COF ⊃ C 60 as an active layer for photoenergy conversion. We selected an organic semiconductor [6,6]-phenyl-C61-butyric acid methyl ester (PCBM) as a glue (50 wt%) to fabricate 1 × 1 cm 2 indium tin oxide (ITO)/active layer/Al cells using spin-coated CS-COF ⊃ C 60 films. The thickness of the active layer was adjusted to ~100 nm. In comparison with PMMA-glued devices, the photocurrents of these film cells were increased by three orders of magnitude. On illumination under air mass 1.5 conditions, the thin film cells exhibited a power conversion efficiency of 0.9% ( Fig. 6f ). The large open-circuit voltage of 0.98 V is remarkable and originates from the low HOMO level (–5.70 eV) of CS-COF. A photovoltaic cell based on thienothiophene-based thieno[2,3-b]thiophene (TT)-COF ⊃ PCBM with a conversion efficiency of 0.053% was reported recently [26] . In the present cell, the COF platelets are not unidirectionally oriented, resulting in boundaries between grains, which interfere with the carrier transport to the electrodes. On the basis of this result, once the present COFs can be obtained as large-area-oriented thin films [25] on transparent electrodes, maximized structural advantages of CS-COFs would be achievable for highly efficient photoenergy conversion. Our findings introduce a new strategy and direction in the quest for three-dimensionally ordered π conjugation polymers. This work describes the first successful synthesis and remarkable property of a chemically stable, electronically conjugated COF that permits inborn periodic structural ordering of conjugated chains in all three dimensions. This new framework has unbroken π-electron conjugation that spans in principle to the entire sheet of COF, a novel combination of excellent physical properties and three-dimensional periodic ordering that typical conjugated polymers are lacking in. The design principle that made this long-pursued achievement possible may guide synthesis of other frameworks that need continuous three-dimensional π-electron conjugation. We anticipate that such conjugated organic zeolites may facilitate innovations and applications in fields from organic electronics to energy storage, and fuel cells. Synthesis of CS-COF A 3-ml pyrex tube was charged with TPHA chloride (16.1 mg, 0.03 mmol), PT (16.8 mg, 0.045 mmol), and 1 ml mixture of ethylene glycol and 3 M acetic acid aqueous solution (1/1 in v/v). The mixture was ultrasonicated for 15 min at 25 °C and degassed using three freeze-pump-thaw cycles. The tube was then sealed and kept in an autoclave at 120 °C for 3 days. The precipitate was filtered off, exhaustively washed by Soxhlet extractions with water, methanol and dichloromethane for 24 h, and was dried at 150 °C under 0.1 Pa for 12 h to yield CS-COF as powders in 86–90% isolation yields. Synthesis of CS-COF ⊃ C60 The thermal sublime diffusion method was employed for loading fullerene into the pores of CS-COF. A mixture of CS-COF and C 60 was placed in a pyrex glass tube and sealed under vacuum. The tube was heated at 400 °C for 50 h and the resultant solid was exhaustively washed with toluene until the liquid phase was colourless. The solid was then dried at 80 °C in vacuum to give CS-COF ⊃ C 60 . Characterization FT IR spectra were recorded on a JASCO model FT IR-6100 IR spectrometer using KBr platelets. Solid-state 1 H or 13 C CP/MAS NMR spectroscopy was carried out using a 920-MHz 1 H NMR spectrometer at a MAS rate of 15 kHz and a CP contact time of 2 ms, and also solid-state 15 N CP/MAS NMR spectroscopy using a 920-MHz 1 H NMR spectrometer at a MAS rate of 30 kHz and a CP contact time of 3 ms with nitromethane as standard. Ultraviolet–visible–IR diffuse reflectance spectrum (the Kubelka–Munk spectrum) was recorded on a JASCO model V-670 spectrometer equipped with integration sphere model IJN-727. Field-emission scanning electron microscope measurements were performed on a JEOL model JSM-6700 operating at an accelerating voltage of 5.0 kV. HR TEM images were obtained on a JEOL model JEM-3200 microscope. The sample was prepared by drop casting a supersonicated acetone suspension onto a copper grid. AFM images were recorded on a Veeco model 3D multimode diNanoScope with samples deposited on mica. XRD data were recorded on a Rigaku model RINT Ultima III diffractometer, from 2 θ =1° up to 60° with 0.02° increment at 25 °C. TGA measurements were carried out on a Mettler Toledo model TGA/SDTA 851e on heating the sample to 1,000 °C at a rate constant of 10 °C min –1 under nitrogen. Gas adsorption Nitrogen sorption was measured at 77 K with a Micromertics Tristar 3000 analyser. Before measurement, the samples were degassed in vacuum at 200 °C for more than 6 h. The Brunauer–Emmett–Teller method was utilized to calculate the specific surface areas. By using the non-local density functional theory model, the pore volume and pore size distribution were derived at a relative pressure P / P 0 <0.1. The calibration curve was obtained by using black carbon (part number 004-16833-00) as a reference material and nitrogen as an adsorption gas. Hydrogen sorption isotherm measurements were carried out on a Hiden Isochema model digital microbalance IGA-002 with sensitivity of 0.1 μg at 77 K. Before the measurements, samples were degassed at 180 °C for 5 h in a high-vacuum system. Computational simulations The molecular structure and electronic properties of monolayer and stacked CS-COF isomers were determined using the DFTB method including the LJ dispersion. The corresponding LJ and crystal-stacking energies as well as the HOMO–LUMO energy gaps were computed. The calculations were carried out with the DFTB+ program package version 1.2 (ref. 61 ). DFTB is an approximate density functional theory method based on the tight binding approach and utilizes an optimized minimal linear combination of atomic orbitals Slater-type all-valence basis set in combination with a two-centre approximation for Hamiltonian matrix elements. The Coulombic interaction between partial atomic charges was determined using the self-consistent charge formalism. The LJ-type dispersion was employed in all calculations to describe van der Waals and π-stacking interactions. The lattice dimensions were optimized simultaneously with the geometry. Standard DFTB parameters for X–Y element pair (X, Y=C, H and N) interactions were employed from the mio-0-1 set http://www.dftb.org . The optimal single-layer 2D model system consisted of 198 atoms for the CS-COF monomer. It had an optimal lattice constant of a = b =29.6 Å. Using the optimized monomer, three different stacking configurations: perfect AA, AA slip-stacked by 0.8 Å in the a and b directions, and AB were optimized. The third dimension of the lattice, c was initialized at 6.25, 6.25 and 5.25 Å for the AA, slipped AA and AB structures, respectively. The interlayer-stacking distances, and the corresponding LJ, and crystal-stacking energies per monolayer of each structure are shown in Supplementary Table S1 . The minimum energy structure for CS-COF is the slipped AA geometry. The final structures had stacking energy of 110.20 kcal mol –1 corresponding to an interlayer distance of 4.01 Å for the CS-COF. HOMO–LUMO gaps for each structure have been also calculated and are shown in Supplementary Table S1 . The CS-COF monolayer has a HOMO–LUMO gap of 2.046 eV and this is not appreciably changed by any stacking configuration, with HOMO–LUMO gaps of 2.013, 2.050 and 1.977 eV for the slipped AA, AA and AB structures, respectively. XRD Pawley refinement Pawley refinement was carried out using Reflex, a software package for crystal determination from XRD pattern, implemented in MS modelling ver 4.2 (Accelrys Inc.) [62] . Unit cell dimension was first manually determined from the observed XRD peak positions by using hexagonal arrangement. Using the obtained information, we performed Pawley refinement to optimize the lattice parameters iteratively until the RWP value converges. The refinement suggests a hexagonal crystal system with a unit cell of α = β =90° and γ =120°, a = b =29.60119 Å and c =3.48934 Å. The pseudo-Voigt profile function was used for whole profile fitting and Berrar–Baldinozzi function was used for asymmetry correction during the refinement processes. The final R WP and R P values were 2.36% and 1.85%, respectively. Simulated XRD patterns were calculated from this refined unit cell and compared with the experimentally observed pattern. Charge carrier mobility measurements Flash photolysis time-resolved microwave conductivity measurements were carried out at 25 °C in Ar or SF 6 where the resonant frequency and microwave power were appropriately adjusted to 9.1 GHz and 3 mW, respectively. Charge carriers were photochemically generated using the third harmonic generation ( λ =355 nm) of a Nd:YAG laser (Spectra-Physics model INDY-HG) with a pulse duration of 3–5 ns. Transient conductivity ( φ Σ μ : the product of the photocarrier generation yield and the sum of the mobilities of the charge carriers) was evaluated using the equation φ Σ μ =(1/A)(Δ P r/ P r), where A and P r are the sensitivity factor and reflected microwave power, respectively. Time-of-flight current transients were measured for the Al/PMMA/Au configuration at 25 °C by photoirradiation from the Au side with the 355-nm pulse laser. The laser intensity was attenuated at 34 mJ cm –2 per pulse, while the bias voltage was 3.5–65 V. For fabrication, CS-COF was homogeneously dispersed in PMMA (CS-COF/PMMA=60/40 in wt%) and cast onto an Al substrate to form an ~1.5-μm-thick film and then overcoated with a 20-nm-thick layer of Au. Photocondctivity measurements Photoconductivity measurements were conducted on CS-COF ⊃ C60 film sandwiched between Al and Au electrodes at 25 °C in air, using a two-probe method with a subfemtoamp sourcemeter (Keithley 6430). For the switch fabrication, CS-COF ⊃ C60 was homogenously dispersed in PMMA (CS-COF ⊃ C60/PMMA=50/50 wt%) and cast onto an Al substrate to give a film with a thickness of 50 nm–100 μm and then overcoated with a 30-nm-thick layer of Au. Light irradiation was performed using xenon lamp (Asahi Spectra model MAX-301). I–V curves were recorded at bias voltages from –2 to 2 V, on irradiation of the Au electrode with the light (>400 nm), while on-off experiments were carried out by on and off the light illumination. Solar cells ITO-coated glass substrates were cleaned by ultrasonication in H 2 O, acetone and 2-propanol. Dispersion of CS-COF ⊃ C60 in N -methyl-2-pyrrolidone was carried out by stirring the solution at 80 °C under Ar for 1 week. A mixture of PCBM in o -dichlorobenzene (40 mg ml –1 ) and the N -methyl-2-pyrrolidone suspension (40 mg ml –1 for CS-COF ⊃ C60) was spin coated (1,000 r.p.m., 30 s) onto ITO substrate. The resulting film on ITO was annealed at 150 °C for 5 min. The thicknesses of the film were checked by AFM measurements and maintained to be about 100 nm. An Al electrode (100 nm) was deposited onto the film under high vacuum. J–V curves of the cells were measured under illumination with a solar simulator air mass 1.5 G. How to cite this article: Guo, J. et al. Conjugated organic framework with three-dimensionally ordered stable structure and delocalized π clouds. Nat. Commun. 4:2736 doi: 10.1038/ncomms3736 (2013).